Emergence of a novel prey life history promotes contemporary sympatric diversification in a top predator Intraspecific phenotypic variation can strongly impact community and ecosystem dynamics. Effects of intraspecific variation in keystone species have been shown to propagate down through the food web by altering the adaptive landscape for other species and creating a cascade of ecological and evolutionary change. However, similar bottom-up eco-evolutionary effects are poorly described. Here we show that life history diversification in a keystone prey species, the alewife ( Alosa pseudoharengus ), propagates up through the food web to promote phenotypic diversification in its native top predator, the chain pickerel ( Esox niger ), on contemporary timescales. The landlocking of alewife by human dam construction has repeatedly created a stable open water prey resource, novel to coastal lakes, that has promoted the parallel emergence of a habitat polymorphism in chain pickerel. Understanding how strong interactions propagate through food webs to influence diversification across multiple trophic levels is critical to understand eco-evolutionary interactions in complex natural ecosystems. Understanding the ecological implications of contemporary evolution is one of the critical challenges for biologists in the twenty-first century [1] , [2] , [3] . It is now well recognized that ecological factors, including human mediated environmental change, can cause rapid evolution, including diversification within species [4] , [5] , [6] . Recent studies have also shown the reciprocal, that the phenotypic variation that emerges on contemporary timescales can have strong effects on ecological processes [1] , [7] , [8] , [9] , [10] . Strong effects of phenotypic variation in predators can propagate down through the food web affecting the ecology of species at multiple lower trophic levels [8] , [9] , [10] , [11] , [12] , and thereby cause a cascade of evolutionary change in prey species [12] . However, to date no such study has empirically addressed the response of higher trophic levels to the divergence of prey on contemporary timescales. For instance, when a prey life history changes due to external events, it is likely that the evolutionary response in the prey alters the adaptive landscape for their predators. Such a change in the adaptive landscape can lead to utilization of and specialization on novel resources and habitats, which may be detected through between-individual differences in foraging ecology and phenotypic traits [13] , [14] . This, in turn, can lead to ecological and/or evolutionary responses, such as diversification, in the predators [15] . Here we ask how contemporary divergence in a keystone prey fish species affects the ecology of a top predator and test the hypothesis that prey divergent evolution can cause diversification in predators using replicate lake ecosystems. Large apex predators have disproportionately large effects on marine, freshwater and terrestrial ecosystems [16] , [17] , [18] with subsequent importance for the ecosystem services that these ecosystems provide humans [19] . Top predators can drive diversification of prey [20] , [21] and help maintain biodiversity [22] . It is typically assumed that apex predators display little phenotypic variation, but there is emerging evidence for rich phenotypic diversity and ecotype formation of predators at the top of multiple food webs [23] , [24] . Yet, the factors promoting this diversity are largely unknown, perhaps because studying large top predators is very difficult on any scale smaller than the whole ecosystem. Most studies of contemporary eco-evolutionary dynamics in multi-trophic communities have been conducted using small scale experiments [9] , [25] , which are powerful tools for testing mechanisms underlying theory, but which cannot test the importance of those mechanisms in natural ecosystems with complex communities [26] . Dammed lakes serve as large-scale experiments of ecological perturbation on natural populations, where barriers to migration force migratory fish into a year-round freshwater life history. Coastal lakes of the North Eastern United States have historically supported large spawning populations of anadromous alewives ( Alosa pseudoharengus ), whose natural life cycle includes a spring spawning run from the ocean through rivers to the lake spawning habitat. Adults usually return to sea shortly after spawning, but juvenile fish remain in the lakes over the summer, where they feed on plankton and grow before migrating to the ocean in autumn [8] . With European colonization of North America, starting ∼ 300 years ago, many streams and rivers were dammed, blocking spawning migration routes and thereby landlocking populations of alewives in dammed lakes [27] , [28] . The year-round presence of these landlocked populations has altered plankton communities [8] , [29] , [30] and alewives have themselves adapted to this modified environment through changes in foraging trait morphology and life history [31] , [32] . In our study lakes, landlocked alewives reside almost exclusively in open-water (pelagic) habitats where they prey upon zooplankton [32] . The ancestral anadromous alewives are found in both pelagic and near-shore (littoral) habitats, where they feed on zooplankton and benthic invertebrates [32] for the duration of their lake residency, ∼ 6 months each year [8] . Alewives are an important food resource for top predators in coastal lakes [33] and, consequently, changes in seasonal availability and habitat use by alewife could affect the ecology and evolution of their predators. The other common prey species that co-occur in coastal lakes are sunfish ( Lepomis spp. ) and yellow perch ( Perca flavescens ), which are primarily found in littoral habitats. The chain pickerel ( Esox niger ), hereafter pickerel, is a native littoral fish predator across their range, and heavily exploits alewife as prey in New England lakes. We hypothesize that contemporary life history changes in alewives in landlocked lakes has created a stable pelagic resource for piscivorous fish, enabling a partial niche shift and phenotypic diversification of the ancestrally littoral pickerel into littoral and pelagic habitat specialists. We test these hypotheses through comparative investigations of population and ecosystem characteristics in multiple New England lakes with either anadromous, landlocked, or no alewife populations ( Fig. 1 ) and analyse pickerel habitat use, short-term (stomach content) and long-term diet (stable isotope-, and C:N ratios), morphology and relatedness along with temporal changes in habitat-specific prey availability. Our analyses show that pickerel have diversified into pelagic and littoral specialists only in the novel lake type, that is, lakes with landlocked alewives and that this diversification is likely caused by a stable high availability of suitable prey fish in the pelagic habitat. 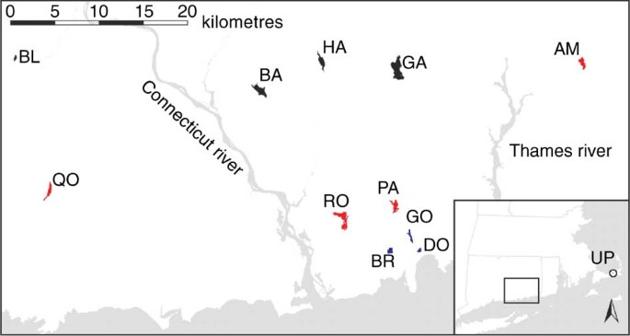Figure 1: Location of study lakes in North Eastern United States. Colours represent lake-type based on absence of alewives (black), and alewife life history (anadromous populations: blue; landlocked populations: red). Most lakes are located in Connecticut (large map), but one lake with an anadromous alewife population is located on Cape Cod, MA (inserted map). Lake names are indicated by abbreviations: Amos Lake (AM), Bashan Lake (BA), Bride Lake (BR), Black Pond (BL), Dodge Pond (DO), Gardner Lake (GA), Gorton Pond (GO), Hayward Lake (HA), Pataganset Lake (PA), Quonnipaug Lake (QO), Rogers Lake (RO) and Upper Mill Pond (UP). Figure 1: Location of study lakes in North Eastern United States. Colours represent lake-type based on absence of alewives (black), and alewife life history (anadromous populations: blue; landlocked populations: red). Most lakes are located in Connecticut (large map), but one lake with an anadromous alewife population is located on Cape Cod, MA (inserted map). Lake names are indicated by abbreviations: Amos Lake (AM), Bashan Lake (BA), Bride Lake (BR), Black Pond (BL), Dodge Pond (DO), Gardner Lake (GA), Gorton Pond (GO), Hayward Lake (HA), Pataganset Lake (PA), Quonnipaug Lake (QO), Rogers Lake (RO) and Upper Mill Pond (UP). Full size image Habitat use We found differences in habitat use (diversification) by pickerel among lakes with anadromous, landlocked and no alewife populations. The use of pelagic habitat by pickerel differed significantly among our three lake types (Pearson χ 2 ( N =42)=12.9; P =0.002; Fig. 2a ), with the occurrence of pelagic pickerel, being significantly more likely in lakes with landlocked alewife than in lakes with anadromous alewife (Pearson χ 2 ( N =26)=4.35; P =0.037) or lakes without alewife (Pearson χ 2 ( N =32)=10.7; P =0.001). Pickerel were regularly caught in the pelagic habitat of lakes with landlocked alewife, but were generally not captured in the pelagic habitat in lakes with anadromous alewives or lakes without alewives, despite similar sampling effort across lakes. The densities of pickerel caught in the littoral habitat also differed among lake types ( F 2,44 =4.17; P =0.025; Fig. 2a ). Differences in littoral densities were due to a lower density of pickerel in lakes without alewives compared with lakes with landlocked alewife (Tukey-HSD( N =30); P =0.01). The density of littoral pickerel in lakes with anadromous alewives was not significantly different from lakes with landlocked alewives (Tukey-HSD( N =30); P =0.56) or from lakes without alewives (Tukey-HSD( N =28); P =0.12). Taken together, these results indicate that pickerel utilize littoral habitats in all lakes, but occupy the pelagic habitat to a much greater extent in lakes with landlocked alewives. 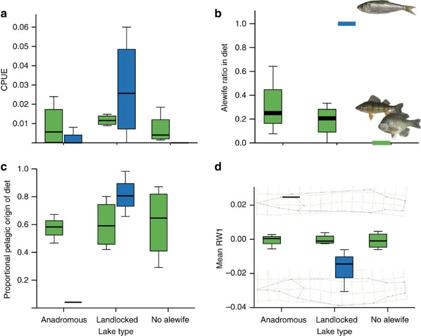Figure 2: Habitat-specific densities and characteristics of chain pickerel in three different lake types based on presence/absence and life history form of alewife populations (anadromous and landlocked). Box plots indicate habitat-specific distribution of lake means with colour indicating habitat type (green: littoral; blue: pelagic) within each lake type. (a) Relative density of chain pickerel. Catch per unit effort (CPUE) refers to number of fish caught per second of electrofishing in the littoral habitat and to number of fish caught per hour per gill net in the pelagic habitat. Densities of pickerel in the pelagic habitat of lakes with landlocked alewives are significantly higher than in the two other lake types and densities in the littoral habitat are lower in lakes without alewives than in lakes with landlocked alewives. (b) Alewife ratio in diet calculated as mean number of alewives/mean number of all prey fish in the diet of chain pickerel. The ratio is significantly higher for pelagic- as compared with littoral pickerel in lakes with landlocked alewives, but do not differ significantly between littoral pickerel from lakes with anadromous and landlocked alewives. (c) Proportional pelagic diet use (α) in chain pickerel calculated from stable isotope analyses (δ13C). Pelagic pickerel had a significantly more pelagic isotope signal than littoral pickerel in lakes with landlocked alewives, whereas there was no significant difference between littoral pickerel from different lake types. (d) Body-depth variation in chain pickerel represented by mean relative warp 1 (RW1). Pelagic and littoral pickerel had significantly different morphology in lakes with landlocked alewives, whereas no significant difference was found between littoral pickerel from different lake types. Note that the figure indicates distribution of lake means, where single values, that is, the single pelagic caught pickerel in lake with anadromous alewives, appear extreme despite being within the range of other values. For all box plots, boxes represent the interquartile range; lines across boxes indicate median values and whiskers extend to the maximum and minimum values. Figure 2: Habitat-specific densities and characteristics of chain pickerel in three different lake types based on presence/absence and life history form of alewife populations (anadromous and landlocked). Box plots indicate habitat-specific distribution of lake means with colour indicating habitat type (green: littoral; blue: pelagic) within each lake type. ( a ) Relative density of chain pickerel. Catch per unit effort (CPUE) refers to number of fish caught per second of electrofishing in the littoral habitat and to number of fish caught per hour per gill net in the pelagic habitat. Densities of pickerel in the pelagic habitat of lakes with landlocked alewives are significantly higher than in the two other lake types and densities in the littoral habitat are lower in lakes without alewives than in lakes with landlocked alewives. ( b ) Alewife ratio in diet calculated as mean number of alewives/mean number of all prey fish in the diet of chain pickerel. The ratio is significantly higher for pelagic- as compared with littoral pickerel in lakes with landlocked alewives, but do not differ significantly between littoral pickerel from lakes with anadromous and landlocked alewives. ( c ) Proportional pelagic diet use ( α ) in chain pickerel calculated from stable isotope analyses ( δ 13 C). Pelagic pickerel had a significantly more pelagic isotope signal than littoral pickerel in lakes with landlocked alewives, whereas there was no significant difference between littoral pickerel from different lake types. ( d ) Body-depth variation in chain pickerel represented by mean relative warp 1 (RW1). Pelagic and littoral pickerel had significantly different morphology in lakes with landlocked alewives, whereas no significant difference was found between littoral pickerel from different lake types. Note that the figure indicates distribution of lake means, where single values, that is, the single pelagic caught pickerel in lake with anadromous alewives, appear extreme despite being within the range of other values. For all box plots, boxes represent the interquartile range; lines across boxes indicate median values and whiskers extend to the maximum and minimum values. Full size image Other piscivorous fish species, all introduced, were never caught in the pelagic habitat in lakes with anadromous alewives, only once in the pelagic of lakes without alewives, but on some occasions in lakes with landlocked alewives. Of the other piscivores besides pickerel, we caught largemouth bass ( Micropterus salmoides ), smallmouth bass ( Micropterus dolomieu ) and walleye ( Sander vitreus ) during the study. All three species are introduced for sport fishing. All smallmouth bass and the far majority of largemouth bass were caught in the littoral habitats of the lakes. Only two largemouth bass were caught in the pelagic habitat, both in a lake with landlocked alewives (Amos Lake). Walleye were only found in two lakes and only in the pelagic habitat (No alewife: Gardner Lake (one individual); landlocked alewife: Rogers Lake (three individuals)). Thus, both pickerel specifically and all piscivores as a group were more abundant in the pelagic habitat of landlocked lakes as compared with the pelagic habitat of other lakes despite that there were no differences in littoral densities of piscivores among lake types. Ecological differentiation Over all lakes, the diet of chain pickerel was composed of 75% fish, 20% crayfish and 5% of smaller invertebrates ( Supplementary Fig. 1 ). Lepomis spp . were the most prevalent fish species in the diet (45–62% between lake types), and alewives, when present in a lake, were the second most prevalent food item (27–35%). Besides these fish species, we found yellow perch ( P. flavescens ), largemouth bass ( M. salmoides ), golden shiner ( Notemigonus crysoleucas ) and rainbow trout ( Oncorhynchus mykiss ) in multiple stomachs and black bullhead ( Ameiurus melas ), black crappie ( Pomoxis nigromaculatus ) and chain pickerel as single occurrences. In lakes with landlocked alewife, pickerel caught in pelagic habitat had a significantly higher proportion of alewife in the diet ( F 1,7 =270.8; P <0.001; Fig. 2b ) and a more pelagic stable isotope signature ( F 1,64 =53.3; P <0.001; Fig. 2c and Supplementary Fig. 2 ), reflecting their almost exclusive diet of pelagic alewife, than the sympatric pickerel caught in the littoral habitat of the same lakes. In contrast, there was no difference in the proportion of alewife in the diet of littoral pickerel from lakes with anadromous and landlocked alewives ( F 1,7 =0.76; P =0.42; Fig. 2b ), and the stable isotope signature of littoral pickerel did not identify any differences in the relative proportion of pelagic diet among lake types (nested ANOVA, F 2,110 =1.86; P =0.16). The single chain pickerel caught in the pelagic habitat in a lake with anadromous alewives did not have a more pelagic signature compared with sympatric littoral caught chain pickerel and, therefore, did not appear to be a habitat specialist. Pickerel also differed in their lipid concentrations, as measured by the C:N ratios of muscle tissue. In lakes with landlocked alewife, pickerel from pelagic habitats had significantly higher lipid concentrations than pickerel from littoral habitats in the same lakes ( F 1,64 =9.9; P =0.003; Supplementary Fig. 3 ). Across lake types, littoral pickerel also differed in lipid concentrations ( F 2,110 =5.5; P =0.006), which was caused by lower lipid concentrations of fish from lakes without alewives compared with lakes with landlocked or anadromous alewife (Tukey-honest significant difference (HSD); P =0.004( N =82) and P =0.081( N =60), respectively). The observed habitat-specific differences in C:N ( Supplementary Fig. 3 ) correspond to a 23% higher mean lipid content in pelagic pickerel (mean±s.d. : 3.1±0.19) as compared with littoral pickerel (mean±s.d. : 2.5±0.14) in lakes with landlocked alewife. The difference in mean C:N for littoral chain pickerel between no alewife lakes and lakes with alewives (either type; Supplementary Fig. 3 ), corresponds to a 23% higher lipid content in littoral chain pickerel from lakes with alewife (either type; mean±s.d. : 2.4±0.26) as compared with littoral pickerel from no alewife lakes (mean±s.d. : 1.9±0.61). The differences in pickerel lipid content are consistent with the much higher lipid content of alewives as compared with bluegill sunfish ( L. macrochirus) , the dominant Lepomis species in most of our study lakes. Morphological diversification In lakes with landlocked alewife, pickerel feeding in pelagic habitats generally showed deeper bodies and more slender heads with shorter upper jaws than pickerel from littoral habitats of the same lakes (relative warp analyses; body: F 1,50 =8.6; P =0.005; Fig. 2d ; head: F 1,50 =6.8; P =0.013; Supplementary Fig. 5A ). In contrast, there were no morphological differences among pickerel found in littoral habitats across the three lake types (body: F 2,98 =0.03; P =0.97; head: F 2,98 =0.77; P =0.47). In each of the three lakes with landlocked alewife populations, where we caught pelagic pickerel, body morphology differed significantly between pelagic and littoral pickerel ( Supplementary Fig. 4 ; Amos Lake: F 1,12 =11.0; P =0.008; Quonnipaug Lake: F 1,15 =5.9; P =0.030; Pataganset Lake: F 1,16 =8.1; P =0.013). Head morphology was significantly different in two of the lakes ( Supplementary Fig. 5B ; Amos Lake: F 1,12 =6.3; P =0.031; Quonnipaug Lake: F 1,15 =6.3; P =0.026), but not in the third (Pataganset Lake: F 1,16 =0.65; P =0.50), which can be ascribed to low sample size of pelagic pickerel in this lake. Origin and relatedness Our microsatellite analyses showed significant genetic differentiation ( F ST ’s) between populations, except between Dodge Pond and Gorton Pond, which are located near each other within the same watershed ( Supplementary Table 1 ). We did not detect any genetic differentiation between pelagic and littoral pickerel within the two tested lakes (Amos Lake and Quonnipaug Lake), but pelagic pickerel were more closely related to littoral pickerel in their own lake than to pelagic pickerel in the other lake or to any other pickerel population ( Supplementary Table 1 and Supplementary Fig. 6 ). Prey availability Prey availability ( F 2,32 =9.9; P =0.027; Fig. 3a ) and temporal stability of the prey resource ( F 2,32 =22.7; P =0.006; Fig. 3b ) in the pelagic habitat varied significantly among lake types for all investigated size classes of pickerel ( Supplementary Fig. 7 ). Post hoc tests showed that prey availability in the pelagic habitat in lakes with landlocked alewife was significantly higher than in lakes without alewife (Tukey-HSD( N =24); P =0.044), and close to significantly higher than in lakes with anadromous alewife (Tukey-HSD( N =20); P =0.069). However, more striking was the much lower seasonal variation in prey availability in the pelagic habitat for all size classes of pickerel in the lakes with landlocked alewife as compared with the two other lake types (Tukey-HSD; P <0.001 for both lakes with anadromous ( N =20) and without alewives ( N =24)), suggesting that prey are not only more abundant in the pelagic of lakes with landlocked alewives than lakes with anadromous or no alewife, but also more stable over the year. 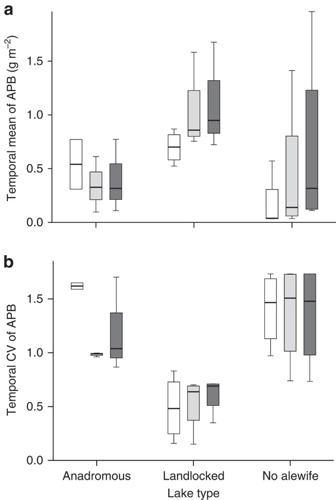Figure 3: Temporal stability in available prey for chain pickerel in the pelagic habitat of three different lakes types based on the presence and life history form of alewives. Pickerel are size selective predators, with an upper and a lower relative size of prey, due to gape-size limitations and relative profitability of prey, respectively. This results in different available prey biomass for different sized individuals occupying the same environment. (a) Available prey biomass (APB) is measured as g m−2and (b) temporal stability in APB as coefficient of variation (CV). Results are indicated for three different size classes of pickerel (white: 300–400 mm; light grey: 400–500 mm; dark grey: 500–600 mm). Available prey biomass varied significantly between lake types, with significantly higher values in lakes with landlocked alewives than in lakes with no alewives (Two-way ANOVA;F2,32=9.9;P=0.027). The temporal stability of the pelagic available prey biomass were significantly higher, that is, lower temporal CV, for the lakes with landlocked alewives than any of the other two lake types (Two-way ANOVA;F2,32=22.7;P=0.006). For all box plots, boxes represent the interquartile range; lines across boxes indicate median values and whiskers extend to the maximum and minimum values. Figure 3: Temporal stability in available prey for chain pickerel in the pelagic habitat of three different lakes types based on the presence and life history form of alewives. Pickerel are size selective predators, with an upper and a lower relative size of prey, due to gape-size limitations and relative profitability of prey, respectively. This results in different available prey biomass for different sized individuals occupying the same environment. ( a ) Available prey biomass (APB) is measured as g m −2 and ( b ) temporal stability in APB as coefficient of variation (CV). Results are indicated for three different size classes of pickerel (white: 300–400 mm; light grey: 400–500 mm; dark grey: 500–600 mm). Available prey biomass varied significantly between lake types, with significantly higher values in lakes with landlocked alewives than in lakes with no alewives (Two-way ANOVA; F 2,32 =9.9; P =0.027). The temporal stability of the pelagic available prey biomass were significantly higher, that is, lower temporal CV, for the lakes with landlocked alewives than any of the other two lake types (Two-way ANOVA; F 2,32 =22.7; P =0.006). For all box plots, boxes represent the interquartile range; lines across boxes indicate median values and whiskers extend to the maximum and minimum values. Full size image Combined, our results suggest the emergence of a novel ecotype of pickerel in lakes with landlocked alewife. The density data indicate greater use of pelagic habitat by pickerel in landlocked lakes and the direct diet data indicate that pickerel are using the pelagic habitat to forage on the landlocked alewife that are found in the pelagic habitat. Our stable isotope results, which provide a long-term integrator of diet, indicate that the pelagic pickerel in landlocked lakes are consistently preying on alewife in the pelagic habitat. The lipid data indicate that the differences in habitat use and diet result in a measureable increase in a component of fitness (lipid storage) for the pickerel in lakes with alewife and a further increase in this fitness component for pickerel feeding almost exclusively on alewife in pelagic habitats. Finally, the morphology data suggest that the pelagic ecotype of pickerel not only feed on different prey, but also have contrasting and potentially adaptive morphology. On the basis of our genetic analyses, we conclude that this differentiation has occurred in parallel, with pelagic pickerel being more closely related to sympatric littoral pickerel than to any allopatric (pelagic or littoral) pickerel. Diversifications in aquatic organisms are often described according to the adaptation to either the pelagic or the littoral habitats (for example, refs 34 , 35 ). These two habitats are often opposite extremes in their structural environment, with the pelagic habitat having no macro-physical structure, whereas the littoral habitat may be highly structured often by plants and rocks. For fish, the adaptation to these different habitats is often associated with morphological divergence related to swimming and feeding performance [36] . The general sagittiform (arrow-like) body shape of pickerel and other esocid fish (family of pikes) is an adaptation to a sit-and-wait foraging strategy, where high strike velocity comes with the cost of less energy efficient continuous swimming [37] . In contrast, a fusiform body shape, characteristic for many pelagic fish species, is an adaptation to energy efficient continuous swimming, which is needed for the ‘pursuit’ hunting behaviour often displayed by pelagic predators. The littoral pickerel of all lakes in the study generally had a maximum body-depth relatively far posterior on their body, which is characteristic for sagittiform fish [38] . In contrast, the pelagic pickerel of landlocked lakes had a maximum body depth further anteriorly and thereby approached a more fusiform body shape. Moreover, the cost of a relatively deeper body shape, as observed in the pelagic pickerel, is expected to be higher drag in burst swimming, whereas the benefit is expected to be higher muscle mass relative to body length. We therefore view the more fusiform and deeper body shape of pelagic pickerel as an expected adaptation to foraging in the pelagic habitat. Likewise, the generally more slender head and shorter upper jaw of the pelagic pickerel is an expected adaptation to feeding on smaller- and more shallow-bodied prey, such as landlocked alewife, compared with the often larger and always deeper-bodied bluegill and perch typically found in littoral habitat. In contrast to the pickerel caught in the pelagic habitat in the landlocked lakes, the single pickerel caught in the pelagic habitat in a lake with anadromous alewives (Bride Lake) had a morphology similar to the littoral pickerel. Hence, in contrast to in landlocked alewife lakes, we did not find a single pickerel in any of the anadromous alewife lakes that was likely to be adapted to the pelagic habitat. The stable isotope and direct diet analyses show clear differences in foraging pattern between pelagic and littoral pickerel, and the higher lipid content of pelagic pickerel suggests the differences in foraging convey a fitness benefit. Small differences in lipid content can have large effects on multiple components of fish fitness, for example, winter survival, reproduction of early spawning fish and growth, when food is not constant. For example, Brodersen et al . [39] showed that winter mortality in a cyprinid fish ( Rutilus rutilus ) were related to a decrease in lipid content of <28% (differences between pelagic and littoral pickerel (in ‘landlocked’ lakes) and between littoral pickerel in different lake types were both 23%). In more lipid-rich fish (for example, rainbow trout [40] ), winter mortality is usually associated with larger proportional decreases in lipid content. Further, esocid females allocate lipids from the relatively lipid-poor muscle tissue into the ovaries, that require a relatively high lipid content [41] . Increased muscle lipid content may, therefore, have an even stronger impact on pickerel fitness through increased reproductive output. A critical question that emerges from these results is why pelagic ecotypes are found only in lakes with landlocked alewives. Since the characteristics of the pelagic habitats do not differ in any other respect than what is associated with life history and presence of alewives [30] , we conclude that the observed diversification in the piscivorous pickerel has been associated with the change in prey life history. More specifically, the availability of fish prey in the pelagic habitat of anadromous lakes was temporally unstable for all sizes of pickerel, with high prey availability for large pickerel at the time of adult alewife spawning migration during late spring, and a high prey availability for small pickerel when juvenile alewives attained sizes available for predation late in the season ( Supplementary Fig. 7 ). In contrast, prey availability for chain pickerel of all sizes in the pelagic habitat of landlocked lakes was much more stable and at a relatively high level throughout the year. The emergence of genetically distinct landlocked alewife populations in New England appears to coincide with colonial dam building [27] . Whereas genetic differentiation has occurred between allopatric populations of pickerel, we did not detect genetic differentiation between co-occurring pairs of littoral and pelagic pickerel within lakes, where we had the largest sample size of pickerel from the pelagic habitat (Amos Lake and Quonnipaug Lake). Spawning segregation within lakes has been found in other esocid species [42] . However, due to the low allele heterogeneity in known microsatellite regions, the relatively low effective population size of top predators, low sample size and the relative short time since emergence of the novel prey phenotypes ( ∼ 300 years) [27] , we may simply not be able to detect assortative mating in the populations. For example, pairwise F ST values were higher between littoral and pelagic pickerel from Amos Lake, where we had the largest sample size, than between allopatric pickerel from Dodge Pond and Gorton Pond ( Supplementary Table 2 ; Supplementary Fig. 6 ), which are both upstream from the same river, but separated by a historical dam. The occurrence of distinct pelagic and littoral pickerel ecotypes could be a result of parallel invasion of a pelagic phenotype evolved in allopatry rather than parallel sympatric diversification in lakes with landlocked alewives. Whereas our preliminary genetic analysis is not strong enough to detect potential genetic differences between littoral and pelagic pickerel within landlocked lakes, it does show that pelagic individuals are more closely related to sympatric littoral individuals than to allopatric pelagic individuals. This suggests that the diversification into pelagic and littoral specialists has occurred in parallel in different lakes with landlocked populations of alewife rather than once, with secondary invasion of pelagic specialists into landlocked lakes. We do not currently know whether the resulting diversity in the pickerel at this early stage of apparent adaptive diversification is heritable or plastic. Regardless, novel niche shifts are a fundamental part of adaptive evolutionary diversification irrespective of whether they are based on plasticity or selection [43] . Whereas novel behavioural niche shifts are necessary for the evolutionary adaptation to a novel niche, the evolutionary adaptation to a novel niche, in return, strengthens behavioural niche shift, giving adapted individuals a higher fitness. Collectively, our results show that a top predator has made a novel niche shift in response to contemporary emergence of a novel prey life history, which, in turn, has promoted parallel ecological and morphological diversification in the top predator. Specifically, the phenotypic divergence of landlocked alewives from their anadromous ancestors, triggered by human dam construction [27] , has yielded a novel seasonally stable niche of pelagic prey for their predators, which in turn promotes predator diversification. This year-round pelagic resource does not occur in lakes with anadromous alewife or in lakes without alewife, which are the two ancestral forms of lakes across Eastern North America. Our findings expand the present understanding of eco-evolutionary interactions by demonstrating that evolution of a novel prey life history can promote diversification in top predators through modified prey availability. Whereas previous research on eco-evolutionary interactions has suggested feedbacks between changes in one organism and its environment [1] , [8] , [11] or its population densities [44] , [45] , the current study extends that perspective by showing that evolutionary changes in one organism may alter the selective landscape for other organisms causing eco-evolutionary interactions to propagate through the food web [12] . Our results also suggest that there may be considerable, but often overlooked, intraspecific variation among top predators. This variation may be of particular importance because of the large impacts top predators have on communities and ecosystems [17] , [18] . Detecting intraspecific variation in wide ranging top predators will, however, require research at large spatial scales and using natural experiments such as those provided by dammed lakes. With the high per-capita impact of top predators on the ecosystem, one of the key questions left to be answered is therefore whether the diversification process in the top predators feedback to strengthen or dampen the diversification process in the prey and how this will further cascade into eco-evolutionary feedback processes at lower trophic levels. Study system Coastal New England lakes harbour either anadromous, landlocked or no populations of alewives, where landlocked populations have diverged from the ancestral anadromous forms in their adaptation to the lake environment [31] , [32] , [46] . We sampled 12 lakes in Connecticut and Massachusetts ( Fig. 1 ; Table 1 ). Four lakes supported large runs of anadromous alewives (Bride Lake, Dodge Pond, Gorton Pond and Upper Mill Pond), four lakes had landlocked alewife populations of independent origin (Pataganset Lake, Amos Lake, Quonnipaug Lake and Rogers Lake) and four lakes did not contain alewife (Black Pond; Bashan Lake, Gardner Lake and Hayward Lake) [8] . All lakes contained piscivorous populations of chain pickerel ( E. niger ) and largemouth bass ( M. salmoides ) and populations of yellow perch ( P. flavescens ), bluegill sunfish ( Lepomis macrochirus ) and pumpkinseed sunfish ( L. gibbosus ). Other fish species varied between lakes, but species composition did not differ significantly between lake types [30] . For a complete list of species in the lakes, see ref. 47 . Lake size ranged from 13.9 to 194.7 ha but did not differ significantly between lake types [8] . Maximum depth varied between 7 and 20 m, except for shallow Gorton Pond (maximum depth 2.5 m), and did not differ significantly between lake types [8] . For further information on lakes see Table 1 . Table 1 Location specific physical and chemical characteristics for the 12 surveyed lakes. Full size table Chain pickerel sampling and density estimation We surveyed each lake during four periods throughout the growing season in 2009, representing different stages in the yearly cycle of alewife life history: May 11–June 1 (anadromous adults present in lakes, but no juveniles); June 15–July 9 (most anadromous adults returned to sea; small juveniles present in lakes); August 10–August 27 (almost solely large juveniles present in anadromous lakes); October 19–November 4 (most juveniles migrated to sea in anadromous lakes). We estimated fish density in both the littoral and in the pelagic habitats, with littoral defined as the near-shore shallow (<2 m) part of the lakes and the pelagic as open water habitats at the deepest part of the lakes. Estimation of fish density was conducted with standardized quantitative electrofishing (Smith-Root SR-16H electrofishing boat; Smith Root, Vancouver, WA, USA) in the littoral habitat and standardized quantitative gill netting in the pelagic habitat. Littoral fish sampling were carried out immediately after sunset in two separate transects representing comparable fractions of stone, sand and vegetation between lakes. Each transect consisted of numerous point samples of active electrofishing, each lasting ∼ 4–10 s adding up to a total of between 111 and 468 s active fishing dependent on fish density. Densities of fish were calculated as number of fish per period of active fishing (see below). Pelagic sampling for piscivores were carried out with five gill nets (length: 38.1 m; height: 1.83 m), each with five different mesh sizes (25.4, 31.8, 38.1, 50.8 and 63.5 mm) in 1.83 m × 7.62 m sections, all targeting relatively large fish. Nets were set 1.5 m below the surface over the deepest part of the lakes in the afternoon and retrieved a few hours after sunset. This period generally covered at least 3 h of daylight and the whole period of civil and nautical twilight. The fishing period ranged from 306 to 527 min (mean±s.d. : 412±47). One lake with anadromous alewives (Gorton Pond) is shallow (maximum 2.5 m) and does therefore not have a pelagic habitat. Instead this pond was sampled with gill nets to test gear selectivity on morphology of chain pickerel (we found no significant difference in stable isotopes or morphology by species caught by gill nets and electrofishing in Gorton Pond). Due to local restrictions on sampling, we did not sample Upper Mill Pond during the first survey and did not use gill nets here during the second survey. No quantitative electrofishing were performed in Bride Lake on the first survey or in Gardner Lake and Black Pond on the fourth survey. To increase sample size for qualitative analyses of morphology, diet content, stable isotope ratios and C:N ratios, we included fish caught with additional electrofishing and beach seining during the survey period ( Supplementary Table 1 ). For analysis of morphology and diet content, we further included chain pickerel caught with gill nets in the littoral during 2006. These fish were, however, not used for stable isotope analyses since reliable baselines were not available for 2006. Whereas the standardized quantitative survey fishing was necessary for comparative density estimates, the supplementary fish were only used in qualitative analyses, for example, between habitats or between lakes, and do therefore not influence quantitative estimates of relative fish densities. The supplementary fish were caught in the same littoral habitats during similar seasons as the fish caught under the standardized quantitative fishing. They were not significantly different in any measures from the fish caught during standardized quantitative fishing and only used to increase accuracy of measurements of population specific estimates of morphology, diet and genotype. We used catch-per-unit-effort (CPUE) as a measure of habitat-specific density of chain pickerel. Since calculations of fish densities can be heavily influenced by high densities of young-of-the-year fish, and since these fish are often not piscivorous, we excluded pickerel <200 mm from the analyses. The 200 mm threshold was chosen as it excludes most young-of-the-year pickerel (92%; Supplementary Fig. 8 ), but includes most 1+ fish (85%; Supplementary Fig. 8 ). We calculated CPUE in the littoral as number of fish caught per second of electrofishing and in the pelagic as number of pickerel caught per net per hour of fishing. Differences in habitat-specific densities between lake types were tested with nested analysis of variances (ANOVAs), with lake nested under lake type and CPUE at each sampling occasion as basic sampling unit. Detailed differentiation between-individual lake types were tested with post hoc tests (Tukey HSD). As pelagic CPUE is often dominated by zeros, which violates the assumptions for the generalized linear model (GLM), we additionally analysed this data using Pearson χ 2 test, where CPUE are translated into presence–absence in a sampling. For each individual fish, length, body mass, muscle tissue sample and stomach content was obtained (for sample sizes, see Supplementary Table 2 ). Due to the relative low numbers in the catch, all pelagic pickerel were sacrificed for morphological analysis whereas only a random subsample of littoral pickerel from each lake was sacrificed for morphological analysis. Fish for morphometric analyses were euthanized with an overdose of MS-222 and individually frozen. Direct diet analyses We obtained stomach content by gastric lavage (as described by Light et al . [48] ) from released fish and by dissection of stomachs from euthanized fish. The gastric lavage method is known to provide close to 100% retention of stomach content [48] , which is also assumed for dissection of stomachs. Stomach content was preserved in 70% ethanol. As pickerels swallow their prey whole, usually head first, most of the observed fish in the stomachs ( n =108 out of n =138: 78%) could be identified to at least genus. Individual prey lengths were obtained for n =110 individual prey fish. Whenever standard length or total length were not obtainable for prey fish, that is, when fish were partly digested, individual length of prey could be estimated from prey specific biometric relationships between caudal fin length and standard length or in a single case where this was not possible, from relationship between height of caudal peduncle and standard length (see Supplementary Table 3 ). We calculated the relative importance of alewife compared with other prey fish, by dividing the mean number of alewives in the diet with the mean number of all identified prey fish in the diet for each habitat in each lake. We analysed differences in diet by t -tests using habitat-specific lake means as sampling unit after arcsine transforming data. Stable isotope and elemental component analyses We estimated the use of pelagic and littoral resources using the stable isotope of carbon ( δ 13 C) using unionid mussels and periphyton as pelagic and littoral end members, respectively [8] , [49] . We used a 6 mm Premier Uni-punch seamless disposable biopsy punch (Delasco, Council Bluffs, IA, USA) to collect a dermal tissue sample from pickerel for stable isotope analysis. Field-collected tissue samples were stored on ice and later frozen. Samples were dried at 55 °C for ∼ 48 h and subsequently ground into a fine powder. One milligram from each sample in tinfoil capsules were analysed on a Europa Geo 20/20 combustion continuous flow isotope ratio mass spectrometer. Each run included a house standard interspersed every 5–9 samples to correct for drift and to provide an estimate of instrumental error. Muscle tissue of brown trout ( Salmo trutta ) from Cayuga Lake, NY, was used as working standard ( δ 13 C=−25.1). Due to low C:N ratios, lipid corrections were not applied [50] (mean±s.d. : 3.17±0.09; maximum value: 3.4). For converting C:N ratios to lipid content, we used the following equation: lipid%=−20.54+7.24 × C:N ratio (ref. 50 ). For baselines in two-end member stable isotope analyses, we collected in all lakes long-lived primary consumers from vegetation or rocks (snails) to provide a littoral end member and from the lake bed (Unionid mussels) for the pelagic end member. We further collected periphyton and zooplankton, that is, short-term baselines, throughout the sample period in all lakes to use as verification of long-term baselines. We sampled periphyton from several rocks from two locations in each lake. We scraped the periphyton off the rocks using toothbrushes and deionized (DI) water and filtered it through a 30-μm mesh and onto pre-ashed Whatman GF-C filters. We took vertical zooplankton hauls with an 80-μm-mesh plankton net from the deepest part of each lake, from approximately one meter below the hypolimnion. Data for mussels, snails, periphyton and zooplankton outside 2 × s.d. from the lake and taxa specific mean were excluded from calculation of lake specific baselines. Relative contribution of pelagic resources in diet ( α ) was calculated from the two-end member-mixing model [49] : where α is the proportion of carbon obtained from the base of food web 1, δ 13 C sc is the stable isotope ratios of the secondary consumer of interest. Our two-end members were the bases of the pelagic and littoral food webs (base1 and base2, respectively). The α -values were constrained to be between 0 and 1. Snails collected were generally very small, shortening the temporal integration [49] , and therefore provided unreliable baselines. Instead of snails, we used the mean δ 13 C-values for periphyton collected over the sampling season as the littoral end members. We were not able to collect any mussels in Black Pond. Here mean δ 13 C-values for zooplankton were used as pelagic baseline. To correct for differences by using zooplankton rather than mussels as pelagic baseline, we corrected this value for Black Pond by the resulting equation from a regression between arcsine transformed mussel periphyton-derived alpha-values ( α asin,MP ) and arcsine transformed zooplankton–periphyton-derived alpha-values ( α asin,ZP ): For all comparative analyses of chain pickerel, we used only data from individuals ≥350 mm, corresponding to the smallest individuals caught in gill nets in the pelagic habitat. This was done to reduce effects of ontogeny from smaller fish that were exclusively caught in the littoral habitat. We tested for differences in stable isotope signature and C:N ratios between pelagic and littoral pickerel in landlocked lakes using an analysis of covariance (ANCOVA) with lake and habitat as independent factors and total length as a covariate; and for differences between littoral pickerel between lake types using a mixed-nested ANCOVA with lake nested under lake type and pickerel total length as co-variable. When the factor ‘lake type’ was significant, we conducted Tukey-HSD post hoc tests without using length as a co-variable. Morphological divergence After thawing, we photographed chain pickerel in the lab for morphological measurements of both whole body and of head shape. Although freezing may potentially have some effects on morphology (see however Valentin et al . [51] ), all individuals were treated equal and if any variation in morphology should be caused by freezing, it would more likely blur differences between ecotypes rather than to falsely indicate them. We used land-marked-based geometric morphometrics for morphological analyses [52] . We digitized 13 homologous landmarks for analysis of body shape and eight for head shape on the left side of the fish ( Supplementary Fig. 9 ) using tpsDig2 software [53] with individuals in random order. The elongated shape of pickerel promotes some bending of the specimens when placed for photography. To reduce the effects of this we statistically unbended all individuals using the unbend-function in the software tpsUtil [53] . For this purpose we used six of the 13 landmarks (as indicated in Supplementary Fig. 9 ). Subsequent analyses, that is, Procrustes fits, partial and relative warp analyses, were performed in the software tpsRelw [53] . Finally, we analysed differences between pelagic and littoral pickerel for individual lakes with landlocked alewife populations using canonical variates analyses using the software MorphoJ [54] , with habitat (littoral versus pelagic) used as classifier variable and 10,000 iterations for permutation test for pairwise distances. While morphological variation shown in relative warp analyses refers to general variation in the global pool of analysed individuals, canonical variates analysis identifies the specific morphological variation associated with different habitats. We only analysed the results from the first relative warp (RW1), as this axis can be taken as predicting the major axis of evolutionary phenotypic divergence among groups, that is, the so-called line of least resistance [55] . RW1 explained 32.2% of the variation in body morphology and 38.2% in head morphology, respectively. We tested for differences in both body and head morphology between pelagic and littoral pickerel in landlocked lakes using an ANCOVA with lake and habitat as independent factors and for differences between littoral pickerel between lake types using a mixed-nested ANCOVA with lake nested under lake type and pickerel total length as co-variable. We only used fish >350 mm in the analyses, corresponding to the size range caught in the pelagic habitat. Fish total length had no effect on body RW1 ( F 1,50 =2.0; P =0.164), but a negative influence on head RW1 ( F 1,50 =6.4; P =0.015). However, as pelagic pickerel in general were slightly larger with more positive RW1 scores, the difference in morphology between littoral and pelagic pickerel was not explained by length. Since length neither influenced body CV1 ( F 1,50 =2.7; P =0.10) nor head CV1 ( F 1,50 =0.03; P =0.88), we did not include length in subsequent lake specific analyses. Hence, we tested for morphological differences (CV1) between littoral and pelagic pickerel in individual lakes with landlocked alewives with simple ANOVAs. Origin and relatedness We tested the genetic relatedness of littoral and pelagic pickerel within and between lakes using analyses of six microsatellite loci. Total genomic DNA was extracted from ∼ 25 mg of frozen muscle tissue using the DNeasy Tissue Kit and animal tissue protocol (Qiagen, Inc., Valencia, CA, USA). We collected genotypic data for the pickerel from seven lakes with landlocked or anadromous alewife populations plus pickerel from the four lakes without alewives. Ten specimens were genotyped per population, except for Bride lake ( N =9), due to low availability of pickerel and Amos Lake ( N =17), where we also attempted tests for spawning segregation between littoral and pelagic pickerel. The genotypic data comprise six microsatellite loci. We used loci initially developed for Esox americanus (EameG12 (forward primer: TCTCTCCCATGCTGAGTGC; reverse primer: ACTGTCTGCCACGACTTCC), EameF07 (forward primer: TGGTCCCCATGAGGTTAGC; reverse primer: CCTTTGCACTTTGGGACTGC), EameA07a (forward primer: TCCTCACTCAAAACCTTCCC; reverse primer: TTCATCCTGGAGGCCACAC), EamP4_B12 (forward primer: CAGACTTCCTAATCGTTTCCTACG; reverse primer: ACAGCATGAATTACCAGAAGAGTG)) and Esox masquinongy (Ema30 (ref. 56 ) and EmaA102 (ref. 57 )). Forward primers were labelled with 6-FAM and HEX fluorescent dyes (Integrated DNA Technologies, Coralville, IA, USA; 6-FAM: EamP4_B12, EameA07a, EameF07; HEX: Ema30, EmaA102, EameG12). We prepared 10 μl reactions using 10–50 ng of template DNA, 5 pmol each of unlabelled reverse and labelled forward primers, 1 × PCR buffer, 25 nmol of MgCl 2 , 2.5 nmol of each dNTP, 1 μg of BSA (New England Biolabs, Ipswich, MA, USA) and 0.5 units of GoTaq DNA polymerase (Promega Corp., Madison, WI, USA). Amplification was carried out via touchdown PCR: initial denaturation at 95 °C for 5 min was followed by reactions cycling through 95 °C, 60 °C to 51 °C (1 °C decrement per cycle) and 72 °C (30 s each), an additional 40 cycles of 95 °C, 50 °C and 72 °C, with a final 20-min extension at 72 °C. PCR products were genotyped on an AB3730xI DNA Analyzer (Applied Biosystems). We used the programme Genemarker v. 1.95 (SoftGenetics, State College, PA, USA) to score the individual genotypes. For allele frequencies see Supplementary Table 4 . We tested for departures from Hardy–Weinberg equilibrium ( Supplementary Table 5 ) and linkage equilibrium ( Supplementary Table 6 ) using a burn-in of 10,000 and 1,000 batches with 10,000 iterations per batch in the programme Genepop v. 4.1 (ref. 58 ). Significance values for multiple comparisons were adjusted using the sequential Bonferroni method [59] . We used the programme Arlequin v. 3.5 (ref. 60 ) to compute summary statistics (allelic richness, observed ( H O ) and expected ( H E ) heterozygosity; Supplementary Table 7 and Supplementary Table 8 ) and also to quantify genetic differentiation via F ST values [61] , the significance of which was tested using 10,000 permutations. The limited population specific sample sizes may cause some noise in the F ST estimates, but are unlikely to cause any directional bias. In order to determine the genetic structure present across the 11 pickerel populations, we subjected the data to both model-based Bayesian clustering, as implemented in Structure 2.3.3 (ref. 62 ), and a multivariate procedure, discriminant analysis of principal components [63] , as implemented in the ‘adegenet’ package [64] in R (ref. 65 ). Structure uses a Markov chain Monte Carlo procedure to group individuals into genetic clusters ( K ) by minimizing deviation from Hardy–Weinberg equilibrium and linkage equilibrium. discriminant analysis of principal components makes no assumptions about Hardy–Weinberg equilibrium and linkage equilibrium and comprises two steps: (1) the principal component analysis step, which reduces the dimensionality of the microsatellite data; and (2) the discriminant analysis step which identifies the linear combination of principal components from the first step that best distinguishes prior groupings, in this case the 11 populations. We used the model with admixture and correlated allele frequencies and performed three independent runs for each K between 1 and 6 using a burn-in period of 50,000 followed by 500,000 Markov chain Monte Carlo steps. We inferred the most probable K both following the suggestions of Pritchard et al . [62] and using the Δ K (second order rate of change) method [66] . Prey availability Habitat- and season-specific prey availabilities were determined in littoral habitats by electrofishing and in the pelagic habitats of all lakes by purse seining. For littoral prey, all fish were collected during electrofishing transects (see above). Pelagic prey abundances were estimated on the first three sampling occasions with purse seining after sunset over the deepest parts of the lakes (for details see Palkovacs et al . [27] ). The purse seining was replicated three times per lake for each sampling day. At the second and third sampling occasion when juvenile alewives were abundant in the pelagic, we counted and released the majority of juvenile anadromous alewives after obtaining a random subsample. This was done since anadromous alewives are a species of concern and measuring all captured alewife would likely have resulted in excessive mortality. The subsample were scooped up with a fine-meshed aquaria net from the aggregated school at the end of the purse procedure. The released fish were counted as they were left to swim out of the purse by a small opening close to the surface under close attention from the field crew. The numbers kept ranged between 168 and 209 (out of totals of between 2,270 and 4,243 corresponding to 4.0–9.2% (except for Dodge Pond where all 455 individuals were kept)) on second sampling occasion and 74 and 87 (out of totals of between 168 and 330 corresponding to 22–52%) at the third sampling occasion. A subset of prey fish from each species were euthanized for biometric analyses (length–body depth–weight relationships; Supplementary Table 3 ). All other fish were measured to the nearest mm (standard length and total length) and released. Optimal prey size was calculated for all lakes combined by regression analysis of biomass of individual prey fish found in pickerel stomachs as a function of individual predator biomass (see below). The relationship between maximum prey body depth (BD) as a function of the chain pickerel length was calculated by a regression of maximum body depth of prey found in pickerel stomachs and chain pickerel total length (assuming intercept=0). Minimum prey size was set to 10% of optimal prey size based on the ‘predation window’ concept [67] , which was in excellent agreement with our empirical data. All were calculated as functions of pickerel body length derived from regression analyses. where m is predator biomass (g) and TL is predator total body length (mm). Available prey biomass was calculated for each sampling period and for each size class of chain pickerel as total biomass of fish between minimum and maximum prey size per sampling effort, that is, surface area of water for purse seining and per minute for electrofishing. Since we calculated available prey biomass for different lengths of pickerel, and both M prey,opt and M prey,min are calculated based on predator body mass, we estimated body mass for the given predator lengths using length weight relationships from all chain pickerel between 300 mm and 600 mm caught during our test fishing in all lakes ( n =192). We analysed differences in prey availability and temporal stability of the prey availability (measured as coefficient of variation) in the pelagic habitat among lakes types for three different size groups of pickerel (300–400 mm; 400–500 mm and 500–600 mm) using two-way ANOVAs with lake type and size group as factors. For prey availability, we used the mean over all sampling periods. Likewise, the temporal stability of the prey availability (CV) was calculated across sampling periods. If interaction between factors was not significant, the analysis was repeated without the interaction term. This study was conducted under our approved Yale University Institutional Animal Care and Use Committee Protocol #2006-10734 and #2009-10734. Fish sampling was conducted under State of Connecticut Scientific Collector Permit #SC-04016, and Commonwealth of Massachusetts collection permit #183.09SCF. How to cite this article: Brodersen, J. et al . Emergence of a novel prey life history promotes contemporary sympatric diversification in a top predator. Nat. Commun. 6:8115 doi: 10.1038/ncomms9115 (2015).